A combinatorial extracellular matrix platform identifies cell-extracellular matrix interactions that correlate with metastasis Extracellular matrix interactions have essential roles in normal physiology and many pathological processes. Although the importance of extracellular matrix interactions in metastasis is well documented, systematic approaches to identify their roles in distinct stages of tumorigenesis have not been described. Here we report a novel-screening platform capable of measuring phenotypic responses to combinations of extracellular matrix molecules. Using a genetic mouse model of lung adenocarcinoma, we measure the extracellular matrix-dependent adhesion of tumour-derived cells. Hierarchical clustering of the adhesion profiles differentiates metastatic cell lines from primary tumour lines. Furthermore, we uncovered that metastatic cells selectively associate with fibronectin when in combination with galectin-3, galectin-8 or laminin. We show that these molecules correlate with human disease and that their interactions are mediated in part by α3β1 integrin. Thus, our platform allowed us to interrogate interactions between metastatic cells and their microenvironments, and identified extracellular matrix and integrin interactions that could serve as therapeutic targets. Cancer metastasis is a poorly understood multistep process that results in 90% of cancer-related deaths [1] , [2] . At the time of initial diagnosis, almost half of lung adenocarcinoma patients have detectable metastases and the majority of the remaining half will relapse with metastatic disease after surgical removal of the primary tumour and adjuvant chemotherapy [3] . Despite the ominous nature of metastatic disease, the molecular mechanisms that drive each step are poorly characterized and few effective therapies exist [4] . Recently, it has become apparent that the tumour microenvironment dramatically impacts metastatic progression [5] . Changes in cancer cell-extracellular matrix (ECM) interactions likely influence each stage of the metastatic cascade, from the loss of basement membrane adhesion to colonization of distant sites. Furthermore, alterations in matrix production and crosslinking can promote metastasis [6] , [7] , [8] . Consequently, inhibiting interactions of tumour cells with their microenvironments by targeting adhesion molecules is an area of active investigation [9] , [10] . Although a variety of techniques exist for studying microenvironmental interactions, it has been challenging to date to interrogate the functional implications of specific cell–ECM interactions in a high-throughput manner. Injection of metastatic cells into embryos documented the anti-tumor effects of the embryonic microenvironment [11] , [12] , and coculture studies have identified the roles of carcinoma-associated fibroblasts on tumour progression [13] . ECM-coated transwells have been used to study the effects of small numbers of individual candidate ECM molecules on 2D invasion [14] , and 3D collagen gels have been useful particularly in the study of matrix metalloproteinase activity [15] . In vivo studies using gene-targeted mice have documented the importance of several ECM molecules and their receptors in transplant-based models of cancer and metastasis [16] , [17] . Each of these techniques has documented key microenvironmental regulators of metastasis, but they have not allowed an unbiased systematic evaluation of the role that ECM components have. Cell–ECM interactions are particularly difficult to study because of their complexity of synergistic and antagonistic interactions in vivo [18] . Experiments targeting integrins, a central family of cell surface receptors that mediate ECM interactions, have implicated integrin–ECM interactions as important regulators of cancer progression [9] , [19] , [20] . However, in addition to adhesion, integrins regulate stress transmission and bidirectional signalling, and typically bind multiple ECM molecules [21] . Furthermore, transmembrane collagens, syndecans, lectins, carbohydrates, gangliosides, glycolipids, CD44 and dystroglycans are among a host of non-integrin ECM receptors. Thus, techniques that allow the specific unbiased interrogation of cell–ECM adhesion are required to directly query the diversity of potential interactions. In this study, we describe a high-throughput platform capable of systematically uncovering cell–ECM interactions, and use this method to characterize the global changes in ECM adhesion in a model of cancer progression. We previously described a first-generation platform that utilized robotic spotting technology to generate arrays with combinations of five ECM molecules found in normal basement membrane and connective tissue [22] . Since then, others have utilized similar platforms to investigate ECM responses [23] , [24] , [25] , [26] . Although these platforms have demonstrated feasibility of such approaches in physiological processes such as differentiation of stem cells, they have not yet been applied to increase our understanding of disease states. Furthermore, their limited size (typically five different ECM molecules) has prevented them from querying the diversity of ECM interactions present in the human body. Here, we present an expanded ECM microarray platform containing 768 unique pairwise ECM molecule combinations expressed differentially in development, regeneration and disease including an expanded representation of proteoglycans and glycosaminoglycans, which are difficult to study through integrin manipulation alone, and apply them to investigate changes in adhesion throughout metastatic progression. We have established a high-throughput pipeline to generate these microarrays that utilizes liquid handlers for mixing of source ECM, optimized cell-seeding devices and automated image capture and analysis. We studied the adhesion profiles of lung adenocarcinoma cell lines generated from a genetically engineered mouse model where discrete stages of metastatic progression have been defined, and correlated the findings with in vivo ECM distributions in mice and humans with metastatic lung cancer [27] , [28] , [29] . This approach is easily extensible to other disease states, ECM combinations and phenotypic readouts. Extracellular matrix microarrays to probe cell–ECM adhesion To allow the unbiased study of the ECM adhesion characteristics of any cells-of-interest, we developed a novel high-throughput platform. We expanded, automated and optimized our adhesion platform [22] , [23] to include every single and pairwise combination of 38 unique ECM molecules ( Supplementary Table S1 ). Thus, these arrays contain 768 different combinations in quintuplicate and 160 control spots, for a total of 4,000 arrayed features. To fabricate the arrays, the 38 ECM molecules and controls are transferred from a 96-well source plate to two low-volume 384-well plates and mixed thoroughly using a robotic liquid handler. These 384-well plates are then used as source plates for deposition of the matrix combinations onto the slides by a DNA microarray spotter. Before deposition of the molecules, slides are coated with a polyacrylamide hydrogel that is allowed to dry after soaking to remove any unpolymerized monomer. The dehydrated hydrogel acts to entrap molecules without requiring their chemical modification ( Fig. 1a ). Our data indicate that molecules larger than ~10 kDa can be robustly entrapped in the hydrogel ( Fig. 1b ), and we verified their entrapment using NHS-Fluorescein labelling or antibody-mediated detection after entrapment ( Fig. 1c ). Of the 38 molecules that we tested by these methods, all showed excellent reproducibility and uniformity within the expected region of printing ( Fig. 1c ). 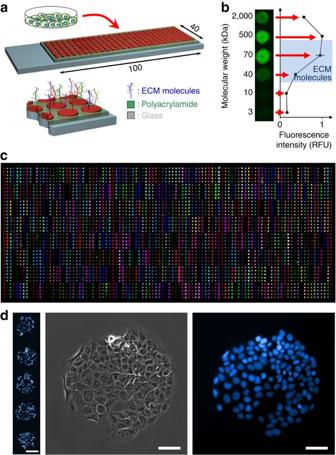Figure 1: Extracellular matrix microarray platform presents combinations of ECM molecules for cell attachment. (a) ECM microarrays are generated by spotting nearly 800 unique combinations of ECM molecules on glass slides coated with polyacrylamide followed by seeding of cells onto the slides. (b) Polyacrylamide acts to entrap molecules of a large range of molecular weights. (c) Verification of presentation of all molecules by immunolabeling (coloured spots) or NHS-fluorescein labelling (grayscale spots) of all molecules subsequent to array generation and rehydration. (d) Representative images of cells adhered to ECM spots demonstrating selective adhesion in the locations of ECM. Scale bar on five-spot image is 200 μm. Scale bars on single-spot images are 50 μm. Figure 1: Extracellular matrix microarray platform presents combinations of ECM molecules for cell attachment. ( a ) ECM microarrays are generated by spotting nearly 800 unique combinations of ECM molecules on glass slides coated with polyacrylamide followed by seeding of cells onto the slides. ( b ) Polyacrylamide acts to entrap molecules of a large range of molecular weights. ( c ) Verification of presentation of all molecules by immunolabeling (coloured spots) or NHS-fluorescein labelling (grayscale spots) of all molecules subsequent to array generation and rehydration. ( d ) Representative images of cells adhered to ECM spots demonstrating selective adhesion in the locations of ECM. Scale bar on five-spot image is 200 μm. Scale bars on single-spot images are 50 μm. Full size image To measure cell–ECM interactions, cells are seeded onto the arrays in serum-free media and allowed to adhere for 1.5 h at 37 °C ( Supplementary Fig. S1a ). To ensure uniform seeding, the slides are agitated every 15 min. Furthermore, the top surfaces of the slides are held flush with the bottom of the plate through the use of a custom-designed seeding device that employs a vacuum seal ( Supplementary Fig. S1b and 1c ). This device minimizes seeding variability between experiments and avoids cell loss by preventing cells from settling below the slide surface or on the backs of the slides. Uniformity of seeding across individual arrays and between replicate arrays was confirmed using test slides composed of only one matrix molecule. To quantify cells bound to each spot, nuclei are stained according to conventional fluorescence staining protocols, and the slides are imaged using an automated inverted epifluorescent microscope with NIS Elements software ( Figs 1 d and 2a ). Large images are cropped to individual spots and indexed using MATLAB (Mathworks), and adhesion is quantified using CellProfiler software to detect and count nuclei ( Fig. 2b ) [30] . Subsequent image and data analysis is performed in MATLAB. 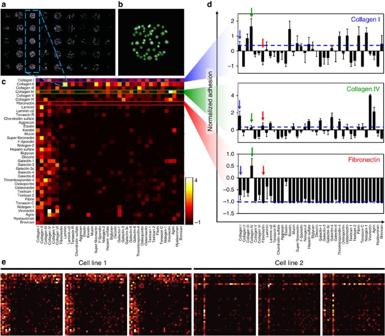Figure 2: Combinatorial adhesion profiles are generated using ECM microarrays. (a) Nuclear stain of cells seeded on the ECM microarrays. (b) Identification of individual nuclei on one spot using CellProfiler30. (c) Quantification of adhesion to all molecule combinations for one cell line. (d) Selected adhesion profiles for three molecules: Collagen I (blue), Collagen IV (green) and Fibronectin (red) in combination with all other molecules. Dashed blue lines represent adhesion to that molecule alone. Arrows denote combinations with the other two molecules or alone. Error bars are s.e.m. of three replicate slides. (e) Comparisons of three replicate slides for two representative cell lines. Scale bars in (a) and (b) are 450 μm and 100 μm, respectively. Figure 2: Combinatorial adhesion profiles are generated using ECM microarrays. ( a ) Nuclear stain of cells seeded on the ECM microarrays. ( b ) Identification of individual nuclei on one spot using CellProfiler [30] . ( c ) Quantification of adhesion to all molecule combinations for one cell line. ( d ) Selected adhesion profiles for three molecules: Collagen I (blue), Collagen IV (green) and Fibronectin (red) in combination with all other molecules. Dashed blue lines represent adhesion to that molecule alone. Arrows denote combinations with the other two molecules or alone. Error bars are s.e.m. of three replicate slides. ( e ) Comparisons of three replicate slides for two representative cell lines. Scale bars in ( a ) and ( b ) are 450 μm and 100 μm, respectively. Full size image ECM microarrays identify distinct adhesion profiles To uncover changes in the global adhesion profile of cancer cells during cancer progression and metastatic spread, we analysed a panel of murine lung adenocarcinoma cell lines derived from non-metastatic primary tumours (T nonMet ), primary tumours that metastasized (T Met ), or lymph node (N) and liver (M) metastases ( Supplementary Table S2 ) [29] . These cell lines were derived from a genetically engineered mouse model of metastatic lung adenocarcinoma in which tumours were initiated in Kras LSL−G12D/+ ;p53 flox/flox mice with lentiviral-Cre vectors. The stable and random integration of the lentiviral vector allowed the clonal relationship between the multifocal primary tumours and metastases to be established [29] . Analysis of the adhesion profiles of these cell lines highlighted the diverse adhesion of each line to different ECM combinations ( Fig. 2c ). Our analysis of these cell lines revealed highly reproducible adhesion between replicate spots and arrays, confirming the quantitative nature of the assay ( Fig. 2e ). We examined the profiles to interrogate whether various populations exhibit enhanced adhesion to combinations of ECM molecules, relative to the same molecules spotted in isolation. This analysis revealed that different pairwise-combinations of ECM molecules result in additive, synergistic and antagonistic effects on adhesion. For example, for the T nonMet cell line shown in Fig. 2c,d , many molecules improve adhesion to collagen I, whereas others reduce cell binding in comparison with the molecule in isolation (blue line, Fig. 2d ). A similar range of responses was observed for other molecules, including collagen IV and fibronectin ( Fig. 2d ). These types of combinatorial effects were present for many molecules, and, while the specific patterns varied, all cell lines tested exhibited examples of increased and reduced binding to various ECM combinations. For each of the 11 murine lung adenocarcinoma cell lines tested, distinct profiles that were highly reproducible across replicate slides were obtained ( Fig. 2e ). We used the ECM microarrays to compare the adhesion profiles of populations from each of the T nonMet , T Met , N and M classes of cell lines. We applied unsupervised hierarchical clustering analysis of the adhesion values in a manner analogous to clustering of gene expression microarray data. Interestingly, all the cell lines derived from metastases (N or M), save for one lymph node line, clustered independently from the cell lines derived from primary lung tumours (T nonMet or T Met ) ( Fig. 3a ). This result is particularly notable, as two of the metastatic lines (393M1 and 389N1) were generated from metastases that originated from two of the primary tumours (393T5 and 389T2, respectively), yet clustered more closely to the other metastases than the lines derived from those primary tumours. Thus, there is a conserved change in the ECM adhesion profile of cancer cells present in a metastatic site versus those that remain in the primary tumour. Furthermore, this differential clustering was not evident from unsupervised hierarchical clustering of the gene expression of these lines (ref. 29 and Supplementary Fig. S2 ), suggesting that the metastasis-specific adhesion phenotype provides a complementary, non-overlapping view of the molecular mediators that influence metastatic progression. 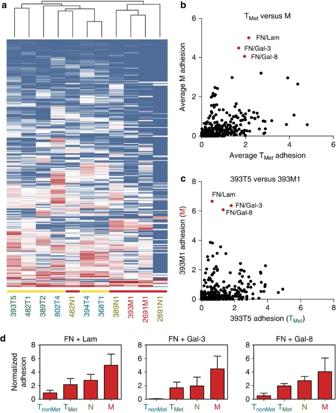Figure 3: ECM microarrays identify key adhesive changes in metastatic progression. (a) Unsupervised hierarchical clustering of adhesion profiles generated by the ECM microarrays. Vertical axis represents different ECM combinations. Horizontal axis represents different cell lines. Yellow bars indicate primary tumours (TnonMetand TMetlines). Red bars indicate nodal (N) or distant metastases (M). (b) Average adhesion of metastatic cell lines (M) to each combination compared with those of the metastatic primary tumour cell lines (TMet). (c) Comparison of 393M1 adhesion for each combination to its matching primary tumour line, 393T5. Red dots indicate top ECM combinations exhibiting preferential adhesion by metastatic lines over the metastatic primary tumour lines. (d) Top three combinations exhibiting the greatest increase in adhesion across tumour progression as represented by the four classes of cell lines (TnonMet, TMet, N and M). Error bars in (d) are s.e.m. of the different cell lines of each class (n=3 cell lines per class) with the exception of the M class where there are two lines, and thus the error bars are the range of the means. Figure 3: ECM microarrays identify key adhesive changes in metastatic progression. ( a ) Unsupervised hierarchical clustering of adhesion profiles generated by the ECM microarrays. Vertical axis represents different ECM combinations. Horizontal axis represents different cell lines. Yellow bars indicate primary tumours (T nonMet and T Met lines). Red bars indicate nodal (N) or distant metastases (M). ( b ) Average adhesion of metastatic cell lines (M) to each combination compared with those of the metastatic primary tumour cell lines (T Met ). ( c ) Comparison of 393M1 adhesion for each combination to its matching primary tumour line, 393T5. Red dots indicate top ECM combinations exhibiting preferential adhesion by metastatic lines over the metastatic primary tumour lines. ( d ) Top three combinations exhibiting the greatest increase in adhesion across tumour progression as represented by the four classes of cell lines (T nonMet , T Met , N and M). Error bars in ( d ) are s.e.m. of the different cell lines of each class ( n =3 cell lines per class) with the exception of the M class where there are two lines, and thus the error bars are the range of the means. Full size image Identification of metastasis-associated ECM molecules In light of the hierarchical clustering results, we asked whether there were particular combinations of molecules that are favored by metastatic cells rather than by cells from primary tumours. Thus, we compared the average adhesion of the liver metastasis-derived cell lines (M) for each ECM combination to the average adhesion of the T Met lines ( Fig. 3b ). Although many of the M lines exhibit elevated binding to combinations containing fibronectin, pairings that combined fibronectin with any of galectin-3, galectin-8 or laminin had the highest differential adhesion between line classes. To explore changes in adhesion that specifically correlated with changes in metastatic progression, we compared the T Met cell line 393T5 and the clonally related liver metastasis-derived cell line 393M1. This pair of lines was derived from a primary tumour and a metastasis that disseminated from that tumour, as confirmed by examination of the lentiviral integration site [29] . Furthermore, the differential adhesion to the aforementioned ECM combinations was clear in both the group-wise comparison ( Fig. 3b ) and in the direct comparison with this primary tumour-liver metastasis pair ( Fig. 3c ). Collectively, the patterns observed suggest that combinations of molecules may have a more significant role in the adhesion profile of a given population than the tendency to bind to any of the ECM molecules alone. Interestingly, the trend towards increased binding to fibronectin/galectin-3, fibronectin/laminin and fibronectin/galectin-8 combinations was consistent across tumour progression when we compared the average adhesion of all T nonMet , T Met , N and M cell lines ( Fig. 3d ). Binding to these molecules, when presented alone, showed minimal (fibronectin) or no trend (laminin, galectin-3 and galectin-8) across the four groups of cell lines ( Supplementary Fig. S3a , red bars). When in combination, however, these pairs demonstrate enhanced effects that exceed the additive values of their individual adhesion. In contrast, other combinations demonstrated a reduced adhesion trend in relatively more metastatic populations, including a variety of collagens and osteopontin ( Supplementary Fig. S3a–c ). Taken together, these data suggest that adhesion to fibronectin in combination with any of galectin-3, galectin-8 or laminin is highly associated with tumour progression in this model system. We also noted that some combinations of molecules appear to elicit antagonistic effects on adhesion. We looked more closely at the adhesion profile of the M line 393M1 ( Supplementary Fig. S4a ) and observed that, whereas the metastasis-associated molecules laminin, galectin-3 and galectin-8 all increase adhesion to fibronectin, other molecules appeared to decrease adhesion to it ( Supplementary Fig. S4b ). In vitro adhesion assays using co-adsorbed ECM to multiwell polystyrene plates confirmed that the addition of these molecules does indeed decrease the adhesion of this line to fibronectin ( Supplementary Fig. S4c ). Collectively, the existence of both synergistic and antagonistic effects highlights the importance of investigating combinations of ECM molecules rather than isolated components. ECM molecules are present in sites of endogenous tumours Next we sought to correlate our in vitro adhesion profiles with ECM expression in vivo . To investigate whether the identified ECM molecules may be important in natural tumorigenesis, organs containing primary autochthonous tumours and their metastases were resected from Kras LSL−G12D/+ ;p53 flox/flox mice and stained. Trichrome staining of lungs with extensive tumour burden revealed a significant presence of ECM deposition in the tumour-bearing lung ( Supplementary Fig. S5a and ref. 31 ). Previously, we found that primary tumours that have acquired the ability to metastasize (T Met tumours) upregulate the chromatin-associated protein Hmga2 (ref. 29 ). Therefore, we used Hmga2 immunohistochemistry in addition to histological characteristics to identify areas of highly aggressive cancer cells ( Supplementary Fig. S5a ). As anticipated, primary lung tumours were positive for collagen I (black arrowheads), collagen VI (open black arrowheads) and osteopontin (red arrowheads), with the most intense staining overlapping with the high-grade tumour areas ( Supplementary Fig. S5a and S5c ). In particular, osteopontin staining strongly co-localized with Hmga2 pos regions, suggesting that increased osteopontin production is associated with metastatic primary lung tumours. Furthermore, little to no laminin, galectin-3 or galectin-8 staining was detected in the primary tumours ( Fig. 4 ). Interestingly, fibronectin staining in the tumour was strong, revealing a correlation between increasingly metastatic populations and the presence of fibronectin early in the metastatic cascade ( Fig. 4 ). 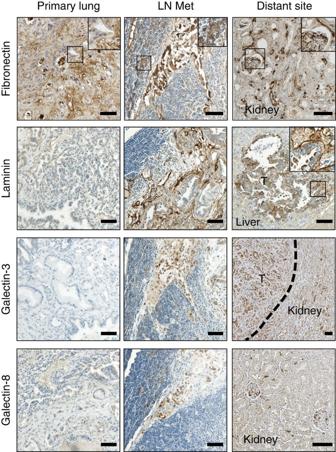Figure 4: Metastasis-associated ECM molecules are present in the sites of metastases but not primary tumours. Immunostaining of the metastasis-associated ECM molecules in the lungs, lymph nodes and distant metastases of mice bearing endogenous lung adenocarcinomas (KrasLSL−G12D/+;p53flox/floxmice). Insets are magnified views of boxed areas showing ECM molecule fibrils. Number of tissues examined for each organ: lungs: 10; lymph nodes: 5; livers/kidneys: 22. 'T': tumour. Dotted line depicts edge of tumour and normal kidney. Scale bars are 50 μm. Figure 4: Metastasis-associated ECM molecules are present in the sites of metastases but not primary tumours. Immunostaining of the metastasis-associated ECM molecules in the lungs, lymph nodes and distant metastases of mice bearing endogenous lung adenocarcinomas ( Kras LSL−G12D/+ ;p53 flox/flox mice). Insets are magnified views of boxed areas showing ECM molecule fibrils. Number of tissues examined for each organ: lungs: 10; lymph nodes: 5; livers/kidneys: 22. 'T': tumour. Dotted line depicts edge of tumour and normal kidney. Scale bars are 50 μm. Full size image We next asked whether the lymph node and distant organ metastases contained the metastasis-associated ECM molecules. Again, trichrome staining revealed the presence of significant matrix deposition within the lymph nodes ( Supplementary Fig. S5b ). As expected, the entirety of the lymph node tumours was histologically high-grade and was Hmga2 pos ( Supplementary Fig. S5b ). There was also clear expression of all four of the metastasis-associated molecules (fibronectin, laminin, galectin-3 and galectin-8) within the lymph node metastases ( Fig. 4 ). Furthermore, there was essentially no collagen I or collagen VI ( Supplementary Fig. S5c ). Osteopontin, however, was present in the metastases ( Supplementary Fig. S5c ) and had its highest expression along the invasive front ( Supplementary Fig. S5a,d ). We also examined common metastatic sites for the presence of the metastasis-associated molecules ( Fig. 4 ). Both galectin-3 and galectin-8 were distinctly visible in these sites. Laminin and fibronectin both appeared to line the sinusoids of the livers of the mice and were also present in the metastases formed there. To determine whether these differences between the primary and metastatic sites were due to altered matrix production by the tumour cells, we performed immunoblots on the 393T5 and 393M1 T Met and M cell lines. Although the M line showed slight increases in fibronectin and laminin production compared with the T Met line, production of both galectins was constant ( Fig. 5a ). Furthermore, collagen I production was constant, and osteopontin production was actually increased in the M line. Taken together, these data suggest that the ECM microarrays identified molecules that were found within the physiologically relevant sites of mice bearing autochthonous tumours, and that production of these molecules is not solely performed by the tumour cells present in those sites. 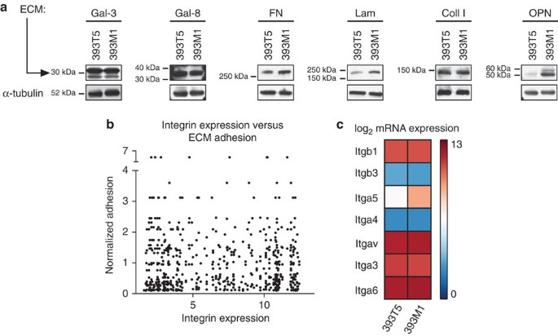Figure 5: ECM production and integrin mRNA expression by cell lines have minimal correlation with adhesion. (a) Western blot analysis of the metastasis- and primary tumour-associated ECM molecules produced by the 393T5 (TMet) and 393M1 (M) cell lines. (b) Comparison of ECM adhesion for all cell lines to gene expression of the cognate integrins from gene expression microarray data. (c) Integrin subunit mRNA expression from Affymetrix microarray analysis in 393T5 and 393M1 cell lines. Figure 5: ECM production and integrin mRNA expression by cell lines have minimal correlation with adhesion. ( a ) Western blot analysis of the metastasis- and primary tumour-associated ECM molecules produced by the 393T5 (T Met ) and 393M1 (M) cell lines. ( b ) Comparison of ECM adhesion for all cell lines to gene expression of the cognate integrins from gene expression microarray data. ( c ) Integrin subunit mRNA expression from Affymetrix microarray analysis in 393T5 and 393M1 cell lines. Full size image Integrin surface expression correlates with ECM-binding profiles We noted that comparisons of adhesion trends on our ECM arrays did not necessarily correlate with transcriptional profiles of the cognate integrins ( Fig. 5b ). Thus, to correlate our findings with the presence of receptors for these metastasis-associated ECM molecules, we examined the clonally related pair of representative T Met and M cell lines for surface expression of their cognate integrins. Although the mRNA expression patterns did not show significant upregulation of the metastasis-associated integrins in the M line by gene expression microarray ( Fig. 5c ), flow cytometry analysis of the integrin subunits corresponding with either the primary tumour-associated molecules or metastasis-associated molecules revealed that the receptor expression trends were consistent with the observed binding patterns. Specifically, integrin subunits known to bind fibronectin (α5 and αv), laminin (α6 and α3) and galectins (α3) were all more prevalent on the metastasis-derived line, while those associated with collagens (α1 and α2) were relatively higher on the primary tumour-derived line ( Fig. 6a ). Nonetheless, the surface expression trends were consistent for the other T Met and M lines as well ( Supplementary Fig. S6a ). Furthermore, within a given cell line, we observed relatively homogeneous surface expression of the metastasis-associated integrins ( Supplementary Fig. S6b ), suggesting that variations in adhesion between lines are due to global increases in surface receptor expression rather than binding patterns of select subpopulations. Immunohistochemistry revealed that these integrins were also present in the metastases of mice bearing autochthonous tumours, but not the adjacent tissue ( Fig. 6b ). The finding that the transcriptional levels of the integrins do not agree with the adhesion trends suggests that post-transcriptional regulation, post-translational modifications such as altered glycosylation or alterations in activation state of the integrins are likely responsible for the changes in adhesion. Thus, by utilizing our platform that investigates specific ECM binding rather than receptor gene or protein expression, we are able to identify candidate ECM interactions that might otherwise have been overlooked. 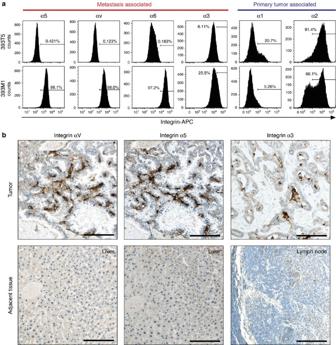Figure 6: Integrin surface expression correlates with ECM-binding profiles. (a) Flow cytometry of integrin surface expression in 393T5 (TMet) and 393M1 (M) cell lines. Integrin subunits that bind to metastasis-associated molecules show increased surface presentation in the metastatic line (α5, αv, α6, α3), while those that bind to primary tumour-associated molecules show decreased presentation (α1 and α2). (b) IHC for metastasis-associated integrins in mice bearing autochthonous tumours with spontaneous metastases to the liver and lymph nodes. Scale bars are 100 μm. Figure 6: Integrin surface expression correlates with ECM-binding profiles. ( a ) Flow cytometry of integrin surface expression in 393T5 (T Met ) and 393M1 (M) cell lines. Integrin subunits that bind to metastasis-associated molecules show increased surface presentation in the metastatic line (α5, αv, α6, α3), while those that bind to primary tumour-associated molecules show decreased presentation (α1 and α2). ( b ) IHC for metastasis-associated integrins in mice bearing autochthonous tumours with spontaneous metastases to the liver and lymph nodes. Scale bars are 100 μm. Full size image Integrin α3β1 mediates adhesion and seeding in vitro and in vivo To examine which candidate receptor/ECM interactions may participate in the observed binding patterns, we performed in silico network mapping of the metastasis-associated ECM molecules using GeneGO software (Metacore) of manually curated molecular interactions. We generated a network map that we termed the lung adenocarcinoma metastasis network that has a greatest disease association with 'Neoplasm Metastasis' ( P =1.094×10 −45 , hypergeometric test, Fig. 7a , Supplementary Fig. S7 ). A network generated using the same parameters but with the primary tumor-associated molecules did not exhibit any disease association with metastasis ( Supplementary Fig. S8 ). Analysis of the lung adenocarcinoma metastasis network identified integrin α3β1 as the surface receptor with the greatest number of edges ( Fig. 7a ). On the basis of this finding, we performed a knockdown of both the α3 and β1 subunits ( Itga3 and Itgb1 , respectively) using short-hairpin-mediated RNA-interference ( Supplementary Fig. S9 ). Knockdown of these genes in the metastatic line, 393M1, resulted in reduced adhesion to the metastasis-associated molecules in vitro when compared with the control hairpin targeting the firefly luciferase gene ( Fig. 7c ). 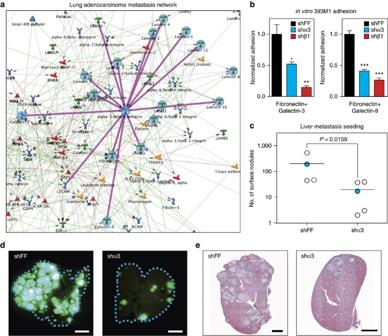Figure 7: Integrin α3β1 mediates adhesion and seedingin vitroandin vivo. (a)In siliconetwork mapping using GeneGO (MetaCore) generates the lung adenocarcinoma metastasis network. Analysis of the network reveals that integrin α3β1 is the surface receptor with the most edges (a). Knockdown of both α3 and β1 integrin subunits by shRNA reduces adhesion to metastasis-associated moleculesin vitro(b) and prevents metastatic seedingin vivo(c–e). shFF is the control hairpin targeting firefly luciferase. One-way ANOVA with Tukey's Multiple Comparison Test was used to analyse the data in figure (b). Error bars in (b) represent s.e. (n=3). (c) Number of liver tumour nodules of the surface of livers 2.5 weeks after intrasplenic injection. Mann–Whitney (non-parametric) test was used to analyse significance. (d) Fluorescence imaging of whole livers after resection. Cell lines express nuclear-excluded ZSGreen. Scale bars are 0.5 cm. (f) Hematoxylin and eosin stain of liver slices. Scale bars are 2 mm. Blue data points in (d) correspond to images in (e) and (f). All results shown are representative of multiple independent experiments. Figure 7: Integrin α3β1 mediates adhesion and seeding in vitro and in vivo . ( a ) In silico network mapping using GeneGO (MetaCore) generates the lung adenocarcinoma metastasis network. Analysis of the network reveals that integrin α3β1 is the surface receptor with the most edges ( a ). Knockdown of both α3 and β1 integrin subunits by shRNA reduces adhesion to metastasis-associated molecules in vitro ( b ) and prevents metastatic seeding in vivo ( c – e ). shFF is the control hairpin targeting firefly luciferase. One-way ANOVA with Tukey's Multiple Comparison Test was used to analyse the data in figure ( b ). Error bars in ( b ) represent s.e. ( n =3). ( c ) Number of liver tumour nodules of the surface of livers 2.5 weeks after intrasplenic injection. Mann–Whitney (non-parametric) test was used to analyse significance. ( d ) Fluorescence imaging of whole livers after resection. Cell lines express nuclear-excluded ZSGreen. Scale bars are 0.5 cm. ( f ) Hematoxylin and eosin stain of liver slices. Scale bars are 2 mm. Blue data points in ( d ) correspond to images in ( e ) and ( f ). All results shown are representative of multiple independent experiments. Full size image We next assessed whether this integrin dimer has a role in metastatic seeding in vivo . Thus, we conducted experimental metastasis assays by intrasplenic injection of 393M1-shα3 or 393M1-shFF cells into wild-type mice, and monitoring for liver tumour formation. We found that mice injected with the 393M1-shα3 cells formed fewer tumour nodules than the controls ( Fig. 7d-f ). Taken together, these findings suggest that the α3β1 integrin dimer has a role in adhesion of metastatic cells to the metastasis-associated ECM molecules and in metastatic seeding. Galectin-3/8 is present in human lung cancer metastases Based on the in vitro adhesion data and in vivo mouse findings, we sought to explore the role of the metastasis-associated ECM molecules in human samples. Using Oncomine [32] , a human genetic dataset analysis tool, we examined the correlation of ECM gene expression and disease severity (for example, clinical stage or the presence of metastases). Results of these queries demonstrate that increased expression of LGALS3 or LGALS8 (galectin-3 and galectin-8, respectively) correlate with increased clinical stage or the presence of metastases ( Fig. 8a ). We next investigated whether galectin-3 protein is present at higher levels in malignant human lung tumours compared with benign non-neoplastic human lung tissue using samples taken from lungs and lymph nodes of patients. Staining for galectin-3 in human tissue microarrays revealed a higher presence of the molecule in lymph nodes of patients with malignant disease (88%) compared with those without cancer (38%) ( Fig. 8b ). Furthermore, there was a higher fraction of galectin-3-positive lymph nodes (88%) than positive primary lung tumour samples (47%), confirming its association with the metastatic site over the primary tumour ( P <0.05, Fisher's exact test). Thus, the ECM microarrays were capable of identifying interactions associated with metastasis in human lung cancer. 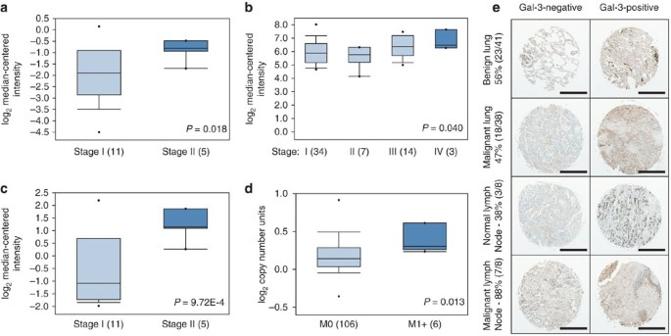Figure 8: Metastasis-associated molecules are present in the metastases of human lung cancers. (a–d) Oncomine32results for human lung cancer expression ofLGALS3andLGALS8. (a)LGALS3Expression in Hou Lung: large cell lung carcinoma—advanced stage. (b)LGALS3expression in Bild Lung: lung adenocarcinoma—advanced stage. (c)LGALS8Expression in Hou Lung: large cell lung carcinoma—advanced stage. (d)LGALS8copy number in TCGA lung 2: lung adenocarcinoma—advanced M Stage.LGALS3andLGALS8are overexpressed in Stage II lung cancer compared with stage I (P=0.018 and 9.72E-4, respectively)(a,c). Microarray data source GSE19188 (ref.46). (b)LGALS3is overexpressed in Stage IV lung cancer compared with other stages (P=0.040). Microarray data source GSE3141 (ref.47). (d)LGALS8has increased copy number in advanced M stage lung cancer (P=0.013) in the 'Lung Carcinoma DNA Copy Number Data' data set available from The Cancer Genome Atlas website (https://tcga-data.nci.nih.gov/tcga/tcgaHome2.jsp). (e) Representative images of human tissue microarray staining results for galectin-3 presence or absence in the primary sites and lymph nodes. Scale bars are 500 μm. Box and whisker plots in (a–d): dots represent maximum and minimum values, whiskers show 90th and 10th percentiles, boxes show 75th and 25th percentiles, and line shows median.P-values in (a–d) were computed by Oncomine software using Student'st-test (a,c,d) or Pearson's correlation analysis (b). Figure 8: Metastasis-associated molecules are present in the metastases of human lung cancers. ( a – d ) Oncomine [32] results for human lung cancer expression of LGALS3 and LGALS8 . ( a ) LGALS3 Expression in Hou Lung: large cell lung carcinoma—advanced stage. ( b ) LGALS3 expression in Bild Lung: lung adenocarcinoma—advanced stage. ( c ) LGALS8 Expression in Hou Lung: large cell lung carcinoma—advanced stage. ( d ) LGALS8 copy number in TCGA lung 2: lung adenocarcinoma—advanced M Stage. LGALS3 and LGALS8 are overexpressed in Stage II lung cancer compared with stage I ( P =0.018 and 9.72E-4, respectively)( a,c ). Microarray data source GSE19188 (ref. 46 ). ( b ) LGALS3 is overexpressed in Stage IV lung cancer compared with other stages ( P =0.040). Microarray data source GSE3141 (ref. 47 ). ( d ) LGALS8 has increased copy number in advanced M stage lung cancer ( P =0.013) in the 'Lung Carcinoma DNA Copy Number Data' data set available from The Cancer Genome Atlas website ( https://tcga-data.nci.nih.gov/tcga/tcgaHome2.jsp ). ( e ) Representative images of human tissue microarray staining results for galectin-3 presence or absence in the primary sites and lymph nodes. Scale bars are 500 μm. Box and whisker plots in ( a – d ): dots represent maximum and minimum values, whiskers show 90th and 10th percentiles, boxes show 75th and 25th percentiles, and line shows median. P -values in ( a – d ) were computed by Oncomine software using Student's t -test ( a , c , d ) or Pearson's correlation analysis ( b ). Full size image Our ECM microarrays provide a high-throughput multiplexed platform capable of measuring a variety of cellular responses to ECM. Here, we show they are capable of identifying adhesion patterns that differentiate metastatic populations from primary tumours. We found that metastatic lung cancer cells preferentially bind to fibronectin in combination with laminin, galectin-3 or galectin-8 compared with cells derived from primary tumours. These changes in adhesion correlate with changes in surface presentation of various integrins. In particular, α3β1 mediates adhesion to these molecules in vitro and permits metastatic seeding in vivo . Furthermore, metastases derived from both a genetically engineered mouse lung cancer model and from human lung cancers express the metastasis-associated ECM molecules. It is worth noting that the combinations of these ECM components elicited the strongest effects, highlighting the importance of using a platform that is capable of measuring responses to more than individual molecules. Galectins are a class of lectins that bind β-galactosides and can associate with other ECM molecules such as fibronectin [33] . Galectin-3 is associated with metastasis in a variety of cancers [34] , [35] and can bind to the oncofetal Thomsen-Friedenreich antigen, a carbohydrate antigen overexpressed by many carcinomas [36] . Our platform confirmed its importance in lung adenocarcinoma, and also identified galectin-8 as having similar importance. Although galectin-8 is known to affect adhesion of cells to other matrix molecules, its role in cancer and metastasis has been less clear as it has been found to have both a positive and negative association with adhesion and tumorigenesis [37] , [38] . Using the ECM microarrays, we showed that binding to galectin-8 in combination with fibronectin is strongly associated with metastatic progression in lung adenocarcinoma. Furthermore, in addition to many collagens, we found that loss of adhesion to osteopontin accompanied metastatic progression ( Supplementary Fig. S3a-c ). Osteopontin levels correlate with prognosis in patients with metastatic disease [39] , and secretion of osteopontin by primary tumours results in mobilization of bone marrow-derived stromal precursors that help establish the metastatic niche [40] . In addition to confirming the presence of the metastatic molecules at the sites of metastases, we found that the invasive portions of primary tumours and the invasive front of the metastases secrete osteopontin ( Supplementary Fig. S5b ). A metastatic tumour line also produces more osteopontin than its corresponding primary ( Fig. 5a ). These findings suggest that while some primary tumours may activate bone marrow cells by secreting osteopontin, in our model, metastatic cells may contribute to this recruitment at a comparable or higher level than the instigating primaries, despite their own loss of adhesion to the immobilized molecule. The use of gene expression signatures for patient stratification in the clinic has become more widespread [41] , [42] , [43] , [44] , [45] , but while genomic approaches have been beneficial for identifying candidate genes, the diversity of findings makes the development of broad therapeutic options seem nearly impossible. By assaying for conserved mechanisms at the phenotypic level, however, relevant targets can be identified and therapeutics can be developed for a broad spectrum of patients. Our results highlight the utility of phenotypic screening approaches for identifying clinical biomarkers. Although we identify α3β1 integrin as a therapeutic target, we also demonstrate that the adhesion signatures generated by the ECM microarrays are capable of differentiating between genetically similar populations with varying metastatic potential. Furthermore, no increase in the mRNA levels of the galectins or their receptors was observed by gene expression microarrays in the M lines ( Fig. 5 and ref. 29 ), despite the association of these molecules with metastasis. The presence of galectin-3 and galectin-8 in human samples ( Fig. 8 ) demonstrates the relevance of this platform to human disease, and thus, we envision that these arrays may be a useful clinical tool for stratification of cancer patients beyond traditional TNM staging. The value of the ECM microarray platform extends beyond the specific application of cancer metastasis. Although this study documents the ability to profile adhesion patterns, cells bound to the arrays can be kept in culture for multiple days to monitor long-term responses to ECM such as cell death, proliferation and alterations in gene or protein expression. Toward that end, one could use multiplexed antibody staining to probe the effects of ECM on stem cell differentiation or activation. Orthogonal screens can be performed to look at the effects of growth factors, small molecules or RNA-interference agents in the context of ECM. Reduction of requisite cell numbers can be achieved using miniaturized arrays to screen rare cell populations such as circulating tumour cells or cancer stem cells and to help expand those populations in vitro for further biological studies. Overall, the ECM microarrays will enhance our ability to study a host of questions as they pertain to both basic biological and clinical settings. Murine lung adenocarcinoma cell lines Cell lines have been described [29] . Briefly, tumour initiation was achieved using intratracheal injection of lentiviral Cre recombinase. Tumours were resected, digested and plated onto tissue culture treated plastic to generate cell lines [29] . Cell lines were subsequently cultured in Dulbecco's modified Eagle's medium (DMEM), 10% foetal bovine serum , penicillin/streptomycin and glutamine. These lines were derived from both primary lung tumours and their metastases. See Supplementary Table S2 for nomenclature regarding cell line origins. Cell transplantation assays All animal procedures were performed in accordance with the MIT Institutional Animal Care and Use Committee under protocol 0211-014-14. Cell injection studies were performed in B6129SF1/J mice (Jackson Laboratory, Stock Number 101043). Intrasplenic injections were performed using 5×10 5 cells resuspended in 100 μl of phosphate-buffered saline (PBS) and injected into the tip of the spleen following existing protocols [29] . Animals were anaesthetized with avertin before surgery. Fur was removed from the animals and they were sterilized with Betadine and 70% ethanol. The spleen was exteriorized following incisions in the skin and body wall. Cells were injected into the end of the spleen with a 27-gauge syringe and allowed to travel into circulation for 2 min. Spleens were then excised from the animals following cauterization of the splenic vessels. The muscle wall was closed using 5-0 dissolvable sutures, and the skin was closed using 7 mm wound clips (Roboz). Mice were killed 2.5–4 weeks following injection, and their livers were excised. Quantification of surface nodules and imaging of livers was performed using a dissection microscope. Tissues were embedded in paraffin following fixation in 4% paraformaldehyde and stained using hematoxylin and eosin. Extracellular matrix microarrays preparation Vantage acrylic slides (CEL Associates VACR-25C) were coated with polyacrylamide by depositing prepolymer containing Irgacure 2959 photoinitiator (Ciba) between the slide and a glass coverslip [22] . Following polymerization, slides were soaked in ddH 2 O and the coverslips were removed. Slides were allowed to dry before molecule deposition. Slides were spotted using a DNA Microarray spotter (Cartesian Technologies Pixsys Microarray Spotter and ArrayIt 946 Pins). 768 combinations were spotted in replicates of five. Rhodamine dextran (Invitrogen) was spotted as negative controls and for use in image alignment. The following molecules were used: Collagen I (Millipore), Collagen II (Millipore), Collagen III (Millipore), Collagen IV (Millipore), Collagen V (BD Biosciences), Collagen VI (BD Biosciences), Fibronectin (Millipore), Laminin (Millipore), Merosin (Millipore), Tenascin-R (R&D Systems), Chondroitin Sulphate (Millipore), Aggrecan (Sigma), Elastin (Sigma), Keratin (Sigma), Mucin (Sigma), Superfibronectin (Sigma), F-Spondin (R&D Systems), Nidogen-2 (R&D Systems), Heparan Sulphate (Sigma), Biglycan (R&D Systems), Decorin (R&D Systems), Galectin 1 (R&D Systems), Galectin 3 (R&D Systems), Galectin 3c (EMD Biosciences), Galectin 4 (R&D Systems), Galectin 8 (R&D Systems), Thrombospondin-4 (R&D Systems), Osteopontin (R&D Systems), Osteonectin (R&D Systems), Testican 1 (R&D Systems), Testican 2 (R&D Systems), Fibrin (Sigma), Tenascin-C (R&D Systems), Nidogen-1 (R&D Systems), Vitronectin (R&D Systems), Rat Agrin (R&D Systems), Hyaluronan (R&D Systems), Brevican (R&D Systems). The laminin used is Millipore catalogue no. AG56P, and is a mixture of human laminins that contain the beta1 chain. Source plates used in the spotter were prepared using a Tecan liquid handler. Molecules were prepared at a concentration of 200 μg ml −1 using a buffer described previously [22] . Slides were stored in a humidity chamber at 4 °C before use. Extracellular matrix microarray seeding and analysis Slides were washed in PBS and treated with UV before seeding cells. They were placed in a seeding device that holds the top surface of the slides flush with bottom of the well. In all, 400,000 cells were seeded on each slide in 6 ml of serum-free medium (DMEM and penicillin/streptomycin). Cells were allowed to attach for two hours at 37 °C. After attachment, slides were washed three times, transferred to quadriperm plates (NUNC, 167063), and new medium was added (DMEM, 10% foetal bovine serum, penicillin/streptomycin and glutamine). Slides were left at 37 °C for two additional hours before removal for staining. Slides were washed twice with PBS and fixed with 4% paraformaldehyde. Nuclei were stained using Hoechst (Invitrogen) in combination with 0.1% Triton-X and PBS. Slides were mounted with Fluoromount-G (Southern Biotech 0100-01) and stored at 4 °C before imaging. Slides were imaged using a Nikon Ti-E inverted fluorescence microscope and NIS Elements Software (Nikon). The entire slide was scanned and images stitched using that software. Image manipulation and analysis was performed in MATLAB (Mathworks) and quantification of nuclei was performed using CellProfiler [30] . Clustering analysis was performed using Spotfire (Tibco). Replicate spots on each slide were averaged and those whose values were >1 s.d. above or below the mean of the replicates were excluded. Slides were normalized to the mean of their non-zero adhesion values. Clustering was performed based on Euclidean distances using Spotfire with the Hierarchical Clustering algorithm (normalized adhesion >0.01). In vitro adhesion seeding In vitro ECM adhesion tests were performed using 96-well-plates (Corning 3603). Plates were coated with 20 μg ml −1 of fibronectin alone or 20 μg ml −1 of fibronectin and 20 μl ml −1 of the second molecule in PBS overnight at 4 °C. Plates were then blocked with 1wt% BSA at room temperature for 1 h. Plates were allowed to dry before adding 2×10 4 cells per well in warm serum-free DMEM. Cells were allowed to adhere for 1 h at 37 °C and shaken every 15 min to ensure uniform seeding. Cells were washed, fixed with 4% paraformaldehyde and stained with Hoechst (Invitrogen). Wells were imaged using a Nikon Ti-E inverted epifluorescent microscope and analysed with Nikon elements software. Protein analysis Western blot analysis of ECM molecules was performed with the following antibodies: galectin-3 (Abcam, ab53082, 1:500), galectin-8 (Abcam, ab69631, 1:500), osteopontin (Abcam, ab8448, 1:2,000), fibronectin (Abcam, ab2413, 1:1,000), laminin (Abcam, b11575, 1:1,000), collagen I (Abcam, ab34710, 1:5,000) and α-tubulin (Cell Signaling, 2125, 1:1,000). Immunohistochemistry of ECM molecules was performed with the following antibodies: galectin-3, galectin-8 (1:75), osteopontin, laminin (Abcam, ab11575, 1:100), fibronectin (Millipore, AB2033, 1:80), Hmga2 (Biocheck, 59170AP, 1:1,000), collagen I (Abcam, ab34710, 1:500) and collagen VI (Abcam ab6588, 1:100). Integrin staining was performed using the following antibodies: integrin αv (Millipore AB1930, 1:200), integrin α5 (Chemicon AB1928, 1:200), integrin α3 antibody was a gift from J.M.L. Tissue microarrays were acquired from LifeSpan Biosciences (LS-SLUCA50), and were stained with the same galectin-3 antibody. Murine tissues were harvested from Kras LSL−G12D , p53 flox/flox mice [27] , [28] , [29] . IHC was performed following resection from mice, fixation in formalin and embedding in paraffin. Flow cytometry analysis of integrin expression was performed using the following antibodies: integrin α5 (Abcam and BioLegend-clone 5H10-27, 1:100), integrin αv (BD-clone RMV-7, 1:100), integrin α6 (BD and BioLegend-clone GoH3, 1:100), integrin α3 (R&D, 1:100), integrin α1 (BD-clone Ha31/8 and BioLegend-clone HMα1, 1:100) and integrin α2 (BD-clone HMα2, 1:100). RNA isolation and expression profiling Cell lysates were harvested using Trizol (Sigma). Chloroform extraction was performed followed by RNA purification using Qiagen RNeasy spin columns. Lysates were analysed for RNA integrity and prepared with Affymetrix GeneChip WT Sense Target Labelling and Control Reagents kit, followed by hybridization to Affymetrix Mouse 3′ Arrays (Mouse 430A 2.0) Lysates used for gene expression microarrays were harvested at the same time as the ECM microarrays were seeded to ensure minimal variability introduced by cell culture. R/Bioconductor software was used to process array images. Unsupervised hierarchical clustering analysis was performed in Spotfire (Tibco) for all probe sets with variance>0.5 and expression>3.0 using Euclidean distances. Data sets are publically available from NCBI under accession number GSE40222 . Retroviral short hairpin RNA (shRNA) constructs miR30-based shRNAs targeting integrins β1 (5′-TGCTGTTGACAGTGAGCGCGGCTCTC AAACTATAAAGAAATAGTGAAGCCACAGATGTATTTCTTTATAGTTTGAGAGCCTTGCCTACTGCCTCGGA-3′), α3 (5′-TGCTGTTGACAGTGAGCGCCGGATGGACATTTCAGAG AAATAGTGAAGCCACAGATGTATTTCTCTGAAATGTCCATCCGTTGCCTACTGCCTCGGA-3′), or control firefly luciferase (5′-AAGGTATATTGCTGTTGACAGTGAGCGAGCTCCC GTGAATTGGAATCCTAGTGAAGCCACAGATGTAGGATTCCAATTCAGCGGGAGCCTGCCTACTGCCTCG-3′) were designed using the shRNA retriever software ( http://katahdin.cshl.edu/homepage/siRNA/RNAi.cgi?type=shRNA ), synthesized (IDT, Coralville, Iowa), and then cloned into the MSCV-ZSG-2A-Puro-miR30 vector [48] . Packaging of retrovirus and transduction of cells was done as described previously [49] . How to cite this article: Reticker-Flynn, N.E. et al . A combinatorial extracellular matrix platform identifies cell-extracellular matrix interactions that correlate with metastasis. Nat. Commun. 3:1122 doi: 10.1038/ncomms2128 (2012).